αE-catenin inhibits YAP/TAZ activity to regulate signalling centre formation during tooth development Embryonic signalling centres are specialized clusters of non-proliferating cells that direct the development of many organs. However, the mechanisms that establish these essential structures in mammals are not well understood. Here we report, using the murine incisor as a model, that αE-catenin is essential for inhibiting nuclear YAP localization and cell proliferation. This function of αE-catenin is required for formation of the tooth signalling centre, the enamel knot (EK), which maintains dental mesenchymal condensation and epithelial invagination. EK formation depends primarily on the signalling function of αE-catenin through YAP and its homologue TAZ, as opposed to its adhesive function, and combined deletion of Yap and Taz rescues the EK defects caused by loss of αE-catenin. These findings point to a developmental mechanism by which αE-catenin restricts YAP/TAZ activity to establish a group of non-dividing and specialized cells that constitute a signalling centre. Epithelial–mesenchymal signalling regulates many developmental processes, including the outgrowth of limbs [1] , the generation of hair follicles and feathers, the budding and branching of developing kidneys, lungs and mammary glands, and the formation of teeth [2] , [3] . Tooth development, which has long served as a model for understanding epithelial–mesenchymal signalling [4] , initiates as the oral epithelium thickenss to become a multilayered structure, known as the placode ( Fig. 1a ). During the transition to the bud stage, the placode first invaginates into the underlying mesenchyme and then undergoes marked morphological changes that result in the formation of two epithelial protrusions at the distal end of the tooth germ, resembling a cap. Concurrently, dental mesenchyme condenses around the epithelium in response to signals from the epithelium. A key event at the bud stage is the formation of a structure called the enamel knot (EK) [5] . In mouse, only one EK is formed in incisors, whereas both primary and secondary EKs are formed in molars. 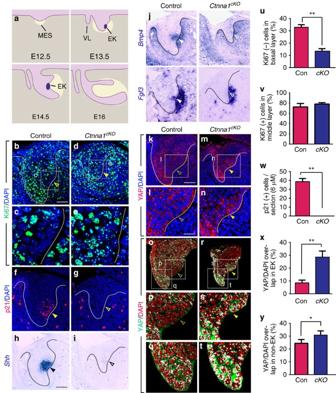Figure 1: Deletion ofCtnna1induces YAP nuclear localization as well as cell proliferation and inhibits EK formation. (a) Schematic diagram of incisor morphogenesis. At E12.5, the dental epithelium (light purple) begins to invaginate into the underlying mesenchyme (MES, tan). By E13.5, the EK is formed. Subsequent epithelial-mesenchymal interactions result in mesenchymal condensation around the epithelium (yellow shaded area). At E14.5, the epithelium turns posteriorly, and the EK regresses by E16. (b,c) At E13.5, the EK consists of post-mitotic cells that are Ki67 negative (open yellow arrowhead). (d,e) Ablation ofCtnna1(Ctnna1cKO) by K14Cre results in ectopic cell proliferation in this region (yellow arrowhead inc). (f,g) p21 is expressed in the control EK (yellow arrowhead) but not inCtnna1cKO(compare yellow arrowhead infto open yellow arrowhead ing). (h–j) EK markers,Shh,Bmp4andFgf3, are absent in theCtnna1cKO(compare black arrowhead inhand white arrowheads injto open black arrowhead iniand open white arrowheads inj). MesenchymalBmp4andFgf3are also reduced. (k,l,o–q) At E13.5, the EK contains mostly cytoplasmic YAP (open yellow arrowheads ink,l), while strong nuclear YAP staining is detected in the surrounding epithelium (q). This is visualized through detection of overlapping signals (white) between YAP (green) and DAPI (red) (open yellow arrowheads ino,p). (m,n,r–t) Deletion ofCtnna1results in YAP nuclear localization in the presumptive EK (yellow arrowheads inm,n,r,s) and the neighbouring epithelium (t). (u,v) Quantification of Ki67-negative (−) cells in the basal layer (u) and Ki67-positive (+) cells in the area surrounding the EK (v) at E13.5 (mean±s.e.m.,n=3,P<0.01). (w) Quantification of p21-positive (+) cells in control andCtnna1cKO(mean±s.e.m.,n=3,P<0.01). (x,y) Quantification of nuclear YAP in the EK region (x) and in the protruding epithelium (y) in control andCtnna1cKO(mean±s.e.m.,n=4,P<0.01 and 0.05 respectively). All quantifications are analysed by using Student’st-test. *P<0.05, **P<0.01. Dotted lines outline the epithelium of the incisor tooth germ. VL, vestibular lamina. Scale bar, 25 μm (b,d,f,g,k,m,o,r); 12 μm (l,n,p,q,s,t); 8 μm (c,e) 50 μm (h,i,j). Figure 1: Deletion of Ctnna1 induces YAP nuclear localization as well as cell proliferation and inhibits EK formation. ( a ) Schematic diagram of incisor morphogenesis. At E12.5, the dental epithelium (light purple) begins to invaginate into the underlying mesenchyme (MES, tan). By E13.5, the EK is formed. Subsequent epithelial-mesenchymal interactions result in mesenchymal condensation around the epithelium (yellow shaded area). At E14.5, the epithelium turns posteriorly, and the EK regresses by E16. ( b , c ) At E13.5, the EK consists of post-mitotic cells that are Ki67 negative (open yellow arrowhead). ( d , e ) Ablation of Ctnna1 ( Ctnna1 cKO ) by K14Cre results in ectopic cell proliferation in this region (yellow arrowhead in c ). ( f , g ) p21 is expressed in the control EK (yellow arrowhead) but not in Ctnna1 cKO (compare yellow arrowhead in f to open yellow arrowhead in g ). ( h – j ) EK markers, Shh , Bmp4 and Fgf3 , are absent in the Ctnna1 cKO (compare black arrowhead in h and white arrowheads in j to open black arrowhead in i and open white arrowheads in j ). Mesenchymal Bmp4 and Fgf3 are also reduced. ( k , l , o – q ) At E13.5, the EK contains mostly cytoplasmic YAP (open yellow arrowheads in k , l ), while strong nuclear YAP staining is detected in the surrounding epithelium ( q ). This is visualized through detection of overlapping signals (white) between YAP (green) and DAPI (red) (open yellow arrowheads in o , p ). ( m , n , r – t ) Deletion of Ctnna1 results in YAP nuclear localization in the presumptive EK (yellow arrowheads in m , n , r , s ) and the neighbouring epithelium ( t ). ( u , v ) Quantification of Ki67-negative (−) cells in the basal layer ( u ) and Ki67-positive (+) cells in the area surrounding the EK ( v ) at E13.5 (mean±s.e.m., n =3, P <0.01). ( w ) Quantification of p21-positive (+) cells in control and Ctnna1 cKO (mean±s.e.m., n =3, P <0.01). ( x , y ) Quantification of nuclear YAP in the EK region ( x ) and in the protruding epithelium ( y ) in control and Ctnna1 cKO (mean±s.e.m., n =4, P <0.01 and 0.05 respectively). All quantifications are analysed by using Student’s t -test. * P <0.05, ** P <0.01. Dotted lines outline the epithelium of the incisor tooth germ. VL, vestibular lamina. Scale bar, 25 μm ( b , d , f , g , k , m , o , r ); 12 μm ( l , n , p , q , s , t ); 8 μm ( c , e ) 50 μm ( h , i , j ). Full size image The EK is composed of a group of densely packed post-mitotic epithelial cells that express the cyclin-dependent kinase inhibitor p21 (p21 Cip1/WAF1 ) [5] , [6] . The principal function of the EK is secretion of an array of signalling molecules, including Sonic hedgehog (SHH), Fibroblast growth factors (FGFs), WNTs and bone morphogenetic proteins (BMPs) [7] , which together regulate tooth morphogenesis. For example, EK-produced FGFs promote cell proliferation both in the mesenchyme and in the epithelium surrounding the EK, driving growth of the tooth germ [8] . EK-produced FGFs also induce expression of FGFs in the adjacent mesenchyme, which reciprocally signal back to the epithelium [9] , driving further development of the tooth. Thus, the EK is considered a signalling centre, and its ability to direct the behaviour of neighbouring cells parallels the function of other developmental signalling centres, such as the apical ectodermal ridge (AER) in the limb bud, the floor plate in the neural tube or the isthmus at the midbrain–hindbrain boundary. However, little is known regarding the molecular mechanism that initiates and maintains signalling centres such as the EK. Histologically, the EK, as well as several other signalling centres such as the floor plate and the isthmus, can be identified as a group of cells with reduced mitotic index [10] , [11] , suggesting that regulated cell proliferation is crucial for their formation and function. The Hippo signalling pathway has been shown to be an important regulator of cell proliferation and differentiation [12] , although little is known about its role in tooth development. The nuclear localization of downstream transcription co-factors, Yes-associated protein (YAP) and its homologue, transcriptional coactivator with PDZ-binding motif (TAZ), allows them to bind to other transcription factors, such as TEAD1-4, and promotes expression of genes that drive cell proliferation [13] . Hippo pathway signalling or other stimuli such as mechanical signalling or increased cell density can lead to phosphorylation of YAP and TAZ by kinases, such as LATS1 and 2, thus rendering YAP and TAZ inactive through sequestration in the cytoplasm and/or degradation [14] , [15] , [16] . A central player that controls YAP/TAZ localization is α-catenin, which retains YAP/TAZ in the cytoplasm as a result of phosphorylation at the S127 site [17] , and deletion of α-catenin can result in uncontrolled YAP accumulation in the nucleus and increased transcriptional activity, driving hyperproliferation in some tissues [17] , [18] . α-catenin is best known for its role as a component of the adherens junction, which also includes cadherins and catenins. In this capacity, α-catenins bind to actin filaments, either directly or through actin-binding proteins, to maintain cellular architecture and seal gaps between neighbouring cells [19] , [20] . In both humans and mice, three α-catenin genes have been identified, Ctnna1 , Ctnna2 and Ctnna3 , which encode αE-catenin, αN-catenin and αT-catenin, respectively. αE-catenin is the most prevalent in epithelial tissues [21] and is required specifically for the morphogenesis of ectodermal appendages. For example, deletion of Ctnna1 with epithelial-specific K14Cre abrogates formation of the hair follicle placodes and sebaceous glands, and loss of Ctnna1 in the mammary gland perturbs cell polarity and differentiation and inhibits alveolar epithelial expansion [22] , [23] . However, the mechanisms by which αE-catenin regulates tissue morphogenesis remain incompletely understood. In this study, we first established that cells within the EK, which are non-proliferating and express high levels of p21, also have low levels of nuclear YAP. By genetically ablating Ctnna1 (encoding αE-catenin) in the dental epithelium, we then showed that αE-catenin is required to prevent nuclear YAP accumulation and ectopic cell proliferation in the EK. Deletion of Ctnna1 thus resulted in loss of the EK, epithelial invagination defects and perturbed mesenchymal condensation. Remarkably, combined deletion of Yap and Taz in the Ctnna1 mutants was able to restore EK formation and rescue the morphogenesis phenotype. These data thus point to a mechanism by which an αE-catenin-YAP/TAZ pathway controls signalling centre formation. The EK has low levels of nuclear YAP The EK is comprised of a group of post-mitotic cells, in contrast to the surrounding epithelium, where active proliferation takes place to support the continuous growth of the tissue [5] . This prompted us to ask whether proper regulation of cell proliferation is required for the formation of the EK. We focused on the incisor because it has a relatively simple structure compared with molars and contains only one EK. As previous experiments mostly investigated development of molars, we first examined cell proliferation in the incisor epithelium by means of Ki67 immunostaining at E13.5, when the formation of the EK is initiated. Similar to the primary EK in the molars, the incisor EK is marked by an area of Ki67 negative cells ( Fig. 1b,c ). This coincides with the expression of the cyclin-dependent kinase inhibitor p21 in the same region ( Fig. 1f ), indicating that EK cells are indeed no longer cycling. Importantly, Shh , Bmp4 and Fgf3 , which are expressed in the molar EK [24] , [25] , [26] , are also expressed in the incisor EK at this stage, providing us additional markers to assess for the presence of these cells ( Fig. 1h,j ). To understand the molecular mechanism that induces cell cycle arrest during formation of the EK, we next examined the expression pattern of the transcription co-factor, YAP, which has been shown to be an important regulator of cell proliferation and differentiation in other tissues [12] . In particular, nuclear YAP promotes the expression of genes that are important for cell proliferation, and its sequestration in the cytoplasm counters that process. In control embryos, consistent with the proliferation profile that was observed in the EK, immunostaining showed nuclear YAP in cells that are located at the protruding lingual and labial tips of the tooth germ, where many cells are proliferating ( Fig. 1k,o,q ). It should be noted that cytoplasmic YAP was also present in these cells, suggesting that a basal level of regulatory control is in place to modulate the amount of YAP inside the nucleus. However, nuclear YAP expression was absent in the EK region, where YAP was mostly localized in the cytoplasm ( Fig. 1k,l,o,p ), consistent with an earlier observation in the molar primary EK [27] . Importantly, the expression patterns of low nuclear YAP, high levels of p21 and low levels of Ki67 observed in the incisor EK were also observed in several other known signalling centres, including the AER, floor plate and isthmus, suggesting that a common mechanism involving YAP may be employed to inhibit cell proliferation within these structures and control their formation ( Supplementary Fig. 1a–x ). 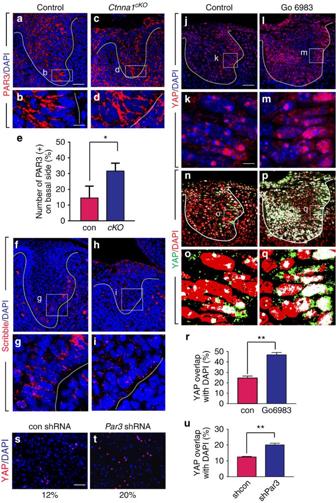Figure 2: αE-catenin is required for maintaining proper cell polarity in the tooth germ epithelium. (a,b) PAR3 is apically localized in cells of the basal layer at E13.5. (c,d) Deletion ofCtnna1causes basal mislocalization of PAR3. (e) Quantification of the cells with mislocalized PAR3 in basal layers of control andCtnna1cKOtooth germs (mean±s.e.m.,n=3,P<0.05). (f,g) Scribble is laterally localized in the basal layer at E13.5. (h,i) The level of Scribble protein is decreased after ablation of αE-catenin. (j–q) Inhibition of aPKC with Gö 6983 induces nuclear localization of YAP in the explant culture. (r) Quantification of nuclear YAP in vehicle and antagonist treated tissues (mean±s.e.m.,n=3,P<0.01). (s,t) Knockdown of PAR3 with shRNA induces YAP nuclear localization in primary epithelial cells. (u) Quantification of nuclear YAP in control (shcon) and shRNA (shPar3)-treated cells (mean±s.e.m.,n=3,P<0.01). All quantifications are analysed by using Student’st-test. *P<0.05, **P<0.01. Dotted lines outline the epithelium of the incisor tooth germ. Scale bar, 25 μm (a,c,f,h,j,l,n,p); 8 μm (b,d,g,i,k,m,o,q); 100 μm (s,t). Figure 2: αE-catenin is required for maintaining proper cell polarity in the tooth germ epithelium. ( a , b ) PAR3 is apically localized in cells of the basal layer at E13.5. ( c , d ) Deletion of Ctnna1 causes basal mislocalization of PAR3. ( e ) Quantification of the cells with mislocalized PAR3 in basal layers of control and Ctnna1 cKO tooth germs (mean±s.e.m., n =3, P <0.05). ( f , g ) Scribble is laterally localized in the basal layer at E13.5. ( h , i ) The level of Scribble protein is decreased after ablation of αE-catenin. ( j – q ) Inhibition of aPKC with Gö 6983 induces nuclear localization of YAP in the explant culture. ( r ) Quantification of nuclear YAP in vehicle and antagonist treated tissues (mean±s.e.m., n =3, P <0.01). ( s , t ) Knockdown of PAR3 with shRNA induces YAP nuclear localization in primary epithelial cells. ( u ) Quantification of nuclear YAP in control (shcon) and shRNA (shPar3)-treated cells (mean±s.e.m., n =3, P <0.01). All quantifications are analysed by using Student’s t -test. * P <0.05, ** P <0.01. Dotted lines outline the epithelium of the incisor tooth germ. Scale bar, 25 μm ( a , c , f , h , j , l , n , p ); 8 μm ( b , d , g , i , k , m , o , q ); 100 μm ( s , t ). 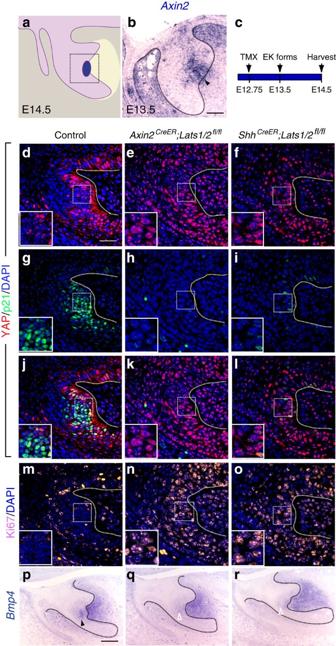Figure 3: Proper YAP localization is essential for the formation of EK during tooth development. (a) Schematic diagram of an E14.5 incisor tooth germ. Square box represents areas imaged ind–o. (b)In situhybridization ofAxin2at E13.5 tooth germ (arrowhead indicates the expression ofAxin2in the EK). (c) Time course for treatment ofAxin2CreER;Lats1/2fl/flandShhCreER;Lats1/2fl/flembryos with tamoxifen to deleteLats1andLats2in the EK. (d,g,j,m) In the EK, YAP is excluded from the nucleus with increased p21 and decreased Ki67 expression at E14.5. (e,f) Double deletion ofLats1andLats2with EK-specificAxin2CreERandShhCreERinduces the nuclear localization of YAP. (h,i) Double deletion ofLats1andLats2with EK-specificAxin2CreERandShhCreERdecreases p21 expression. (k,l) Overlay images of YAP and p21 staining. (n,o) Double deletion ofLats1andLats2in the EK induces ectopic cell proliferation, as shown by Ki67 staining. (p)In situhybridization of the EK markerBmp4at E14.5 (black arrowhead). (q,r) Double deletion ofLats1andLats2inhibitsBmp4expression (open white arrowheads). Dotted lines outline the tooth germ epithelium inb–r. Scale bar, 50 μm (b,c); 25 μm (d–o); 100 μmp–r). Full size image Figure 3: Proper YAP localization is essential for the formation of EK during tooth development. ( a ) Schematic diagram of an E14.5 incisor tooth germ. Square box represents areas imaged in d – o . ( b ) In situ hybridization of Axin2 at E13.5 tooth germ (arrowhead indicates the expression of Axin2 in the EK). ( c ) Time course for treatment of Axin2 CreER ;Lats1/2 fl/fl and Shh CreER ;Lats1/2 fl/fl embryos with tamoxifen to delete Lats1 and Lats2 in the EK. ( d , g , j , m ) In the EK, YAP is excluded from the nucleus with increased p21 and decreased Ki67 expression at E14.5. ( e , f ) Double deletion of Lats1 and Lats2 with EK-specific Axin2 CreER and Shh CreER induces the nuclear localization of YAP. ( h , i ) Double deletion of Lats1 and Lats2 with EK-specific Axin2 CreER and Shh CreER decreases p21 expression. ( k , l ) Overlay images of YAP and p21 staining. ( n , o ) Double deletion of Lats1 and Lats2 in the EK induces ectopic cell proliferation, as shown by Ki67 staining. ( p ) In situ hybridization of the EK marker Bmp4 at E14.5 (black arrowhead). ( q , r ) Double deletion of Lats1 and Lats2 inhibits Bmp4 expression (open white arrowheads). Dotted lines outline the tooth germ epithelium in b – r . Scale bar, 50 μm ( b , c ); 25 μm ( d – o ); 100 μm p – r ). Full size image αE-catenin regulates YAP localization in the EK The results above led us to hypothesize that the exclusion of YAP from the nucleus may be a mechanism for establishing a group of non-proliferating cells that become specialized in signal production within a growing tissue. To test this, we set out to perturb YAP localization. As cytoplasmic retention of YAP depends on the presence of αE-catenin [17] , we first asked whether absence of αE-catenin would increase nuclear YAP. We genetically deleted Ctnna1 , which encodes αE-catenin, in the dental epithelium by crossing a conditional allele of Ctnna1 ( Ctnna1 fl/fl ) with Keratin 14 Cre ( K14 Cre ) [28] , [29] , where Cre recombinase is regulated by the K14 promoter and is expressed in the oral epithelium starting at E11.75, enabling deletion of αE-catenin throughout the entire tooth germ epithelium ( Fig. 4a–d ). Loss of Ctnna1 resulted in YAP accumulation in the nucleus in the presumptive EK region ( Fig. 1m,n,r,s ). This increase in nuclear YAP paralleled what has been observed in the epidermis after deletion of αE-catenin [17] . Quantification of overlapping signals between YAP and nuclear DAPI further confirmed that αE-catenin loss led to nuclear YAP in the region that would form the EK in controls ( Fig. 1x ). Using Student’s t -test, we observed a statistically significant increase of nuclear YAP in the protruding dental epithelium adjacent to the EK as well ( Fig. 1t,y ), suggesting that αE-catenin also inhibits YAP accumulation in these cells. Interestingly, proliferation in non-EK epithelial cells was not affected by Ctnna1 deletion ( Fig. 1v ), most likely because nuclear YAP is normally present in these cells and a further increase in nuclear YAP had limited effects on cell cycle regulation. 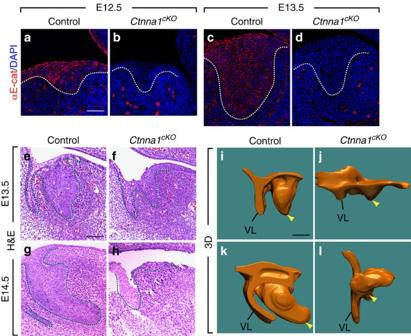Figure 4: αE-catenin is required for incisor epithelium invagination. (a–d) αE-catenin is normally expressed throughout the dental epithelium at E12.5 and E13.5, but expression is absent inCtnna1cKO. (e–l) Histological analysis and 3D reconstruction show smaller and abnormally shaped tooth germs at E13.5 and developmentally arrested epithelia at E14.5 inCtnna1cKO(f,h,j,l) when compared with littermate controls (e,g,i,k). Dotted lines outline the tooth germ epithelium ina–h, and yellow arrowheads indicate the tooth germ epithelium ini–l. VL, vestibular lamina. Scale bar, 25 μm (a–d); 100 μm (e–h); 200 μm (i–l). Figure 4: αE-catenin is required for incisor epithelium invagination. ( a – d ) αE-catenin is normally expressed throughout the dental epithelium at E12.5 and E13.5, but expression is absent in Ctnna1 cKO . ( e – l ) Histological analysis and 3D reconstruction show smaller and abnormally shaped tooth germs at E13.5 and developmentally arrested epithelia at E14.5 in Ctnna1 cKO ( f , h , j , l ) when compared with littermate controls ( e , g , i , k ). Dotted lines outline the tooth germ epithelium in a – h , and yellow arrowheads indicate the tooth germ epithelium in i – l . VL, vestibular lamina. Scale bar, 25 μm ( a – d ); 100 μm ( e – h ); 200 μm ( i – l ). Full size image αE-catenin-mediated cell polarity regulates YAP localization Our observation that loss of αE-catenin leads to increased nuclear YAP is consistent with earlier findings [17] . While this could be in part due to loss of the interaction between YAP and αE-catenin through 14-3-3 binding [17] , deletion of αE-catenin may also result in perturbed cell polarity, which has been recently shown to play a role in regulating YAP distribution [30] , [31] , [32] . To address this possibility, we first examined whether cell polarity is affected in the Ctnna1 mutants by assessing the expression pattern of PAR3 and Scribble, which are markers of apical–basal and basal–lateral polarity, respectively. In the control tooth germ at E13.5, the basal epithelial layer is distinctly polarized, as indicated by the presence of PAR3 on the apical side ( Fig. 2a,b ) and Scribble on the lateral surface ( Fig. 2f,g ). In contrast, in the Ctnna1 mutants, PAR3 was no longer apically restricted, and Scribble expression was largely downregulated ( Fig. 2c–i ). These results indicate that cell polarity was disrupted in the absence of αE-catenin and point to the possibility that mislocalization of YAP in Ctnna1 mutants could be attributable to the loss of cell polarity. To test this hypothesis, we utilized the tooth explant culture system, which is a classical method for maintaining developing tooth germs in vitro [33] and allows functional studies using chemical inhibitors. We disrupted the PAR/aPKC pathway that is essential for the formation and maintenance of cell polarity [34] by inhibiting aPKC with the addition of Gö 6983 (ref. 35 ). This led to increased nuclear YAP in the presumptive EK region after 3 days of culturing ( Fig. 2l,m,p–r ), in contrast to the control tooth germs cultured with dimethyl sulfoxide (DMSO) vehicle, where low nuclear YAP was observed in the EK ( Fig. 2j,k,n,o,r ). Inhibition of Par3 expression with shRNA virus in primary dental epithelial cells also increased YAP nuclear localization in vitro ( Fig. 2s–u ). These results are consistent with the notion that cell polarity is critical for YAP regulation and provide further information regarding control of YAP localization by αE-catenin. αE-catenin is required for EK formation As nuclear YAP is associated with cell proliferation, we next studied whether this increase in nuclear YAP in the posterior region of the tooth germ epithelium leads to ectopic cell proliferation in Ctnna1 cKO by performing Ki67 staining. We examined E13.5 tooth germs, in which the early stages of the EK can be identified as a Ki67 negative non-proliferating zone at the posterior region of the control tooth germ epithelium ( Fig. 1b,c ). However, in the E13.5 Ctnna1 cKO , ectopic cell proliferation was found in this region ( Fig. 1d,e,u ), which suggested that the EK was not forming. To further assess EK formation, we examined the expression of p21. At E13.5, when the EK is first formed, robust p21 immunostaining was observed in the control EK ( Fig. 1f ). In contrast, no p21-positive cells were observed in the Ctnna1 cKO incisor epithelium ( Fig. 1g,w ). Consistent with this result, in situ hybridization of three additional EK markers, Shh , Bmp4 and Fgf3 , confirmed the absence of the EK ( Fig. 1g,j ). These results suggested that YAP might function downstream of αE-catenin to induce cell proliferation and inhibit EK formation. To test this hypothesis, we took advantage of a constitutively active Yap allele ( Yap S127A ) [17] , which is under the control of a tetracycline promoter. When crossed to a Cre allele in conjunction with a Cre-responsive tetracycline activator (ROSA26-rtTA) [36] , conditional expression of Yap S127A can be achieved by administering tetracycline to the animal. When we drove expression of Yap S127A in the incisor epithelium using K14 Cre , a high level of nuclear YAP was detected in about 80% of the cells in the epithelium ( Supplementary Fig. 2a,b ). The incomplete activation of nuclear YAP is likely the result of phosphorylation of the remaining serine sites in YAP S127A , rendering the protein still liable for degradation. Nonetheless, by means of Student’s t -test, we observed a significant downregulation of p21 expression and an increase in Ki67 expression in the EK region ( Supplementary Fig. 2c–j ). These results indicate that expression of active YAP phenocopies some aspects of the Ctnna1 cKO incisor phenotype and demonstrate that nuclear YAP increases cell proliferation and inhibits EK formation. However, the residual EK was sufficient to enable further development of the Yap S127A tooth germ, such that incisor development was relatively normal at later stages, although the protrusion of cells on the lingual aspect seemed to be delayed ( Supplementary Fig. 3 ). We next tested the effect of activation of nuclear YAP specifically in the EK region. To do this, we utilized Axin2 CreER , as Axin2 is highly expressed in the EK at E13.5 ( Fig. 3b ), to generate Axin2 CreER ; Lats1 fl/fl ; Lats2 fl/fl ( Lats1/2 cKO ) embryos, where Cre recombination of Lats1/2 is induced in the EK by delivery of tamoxifen at E12.75 ( Fig. 3c ). This strategy allowed better temporal control compared with the Yap S127A allele, which requires administration of both tamoxifen and doxycycline for activation. In addition, as LATS1/2 phosphorylate most of the serine phosphorylation sites on YAP including S127, deletion of Lats1/2 should result in more robust nuclear YAP localization than Yap S127A misexpression in the EK, due to increased YAP stabilization. Indeed, we observed elevated nuclear YAP in the Lats1/2 cKO EK region at E14.5, 42 h after tamoxifen injection (compare Fig. 3e,k with Fig. 3d,j ). In response to this, p21 expression was downregulated and Ki67 became apparent in the presumptive EK region (compare Fig. 3h,k,n with Fig. 3g,j,m ), consistent with the Ctnna1 cKO phenotype ( Fig. 1d,e,g ). Morphologically, Lats1/2 cKO also lost the characteristic bulge of the EK ( Fig. 3j,k ). To definitively confirm loss of the EK at E14.5, we performed Bmp4 in situ hybridization. Both Shh and Fgf3 are not adequate markers at this stage, as Shh expression is no longer restricted to the EK, while Fgf3 expression is much reduced. In agreement with the p21 and Ki67 expression, the level of Bmp4 expression was decreased in the Lats1/2 cKO EK region ( Fig. 3p,q ). A similar result was obtained when using Shh CreER ( Fig. 3f,i,l,o,r ), which was also highly expressed in the EK region ( Fig. 1h ). Interestingly, the development of the tooth germ was largely normal in both cases, which is likely because both Axin2 CreER and Shh CreER only become active during or right after the EK has formed, resulting in a relatively normal EK at E13.5 ( Supplementary Fig. 4 ), which was not maintained at E14.5 following Lats1/2 deletion and YAP accumulation in the nucleus. αE-catenin is required for incisor morphogenesis To further investigate how deletion of Ctnna1 and the subsequent loss of EK affect tooth development, we next characterized phenotypes associated with the epithelium itself by means of hematoxylin and eosin (H&E) staining. Such histological analysis showed that although no discernible differences were observed at E12.5 ( Supplementary Fig. 5g,h ), the dental epithelium was smaller in all mutants at E13.5 ( Fig. 4e,f ), when a range of abnormal phenotypes was observed. These phenotypes fell into three groups: a bud that lacks distinct lingual and labial tips (39%); a bud with a narrow body that tapers into a sharpened labial end but no obvious lingual protrusion (25%); or a bud with a narrow body and a rounded labial end (36%) ( Supplementary Fig. 5a–d ). By E14.5, growth of the tooth germ was arrested and further invagination did not occur ( Fig. 4g,h ). By E16.5, the incisor was absent in all αE-catenin mutants ( Supplementary Fig. 5e,f ). Three-dimensional (3D) reconstruction of the tooth germ epithelium provided a more comprehensive view of these defects. While the control epithelium at the posterior side began to protrude when turning posteriorly at E13.5 ( Fig. 4i ), the mutant dental epithelium appeared smaller and no posterior turning was observed ( Fig. 4j ). By E14.5, only a small epithelial remnant could be seen in Ctnna1 cKO ( Fig. 4l ), contrasting markedly with the control epithelium, where epithelial invagination continued and the anterior–posterior asymmetry became even more pronounced ( Fig. 4k ). This reduction in the size of the incisor epithelium was not caused by changes in cell death, as detection of apoptosis using TUNEL staining showed no difference between control and Ctnna1 cKO ( Supplementary Fig. 5q,r ). In addition to the invagination phenotype, we also observed that cells were often lost on the oral surface and gaps could be seen within the epithelium of the Ctnna1 cKO ( Fig. 4f,h and Supplementary Fig. 5b–d ), suggesting reduced cell–cell contact consistent with the role of αE-catenin as a key component of the adherens junction. To test whether adherens junctions were affected in the absence of αE-catenin, we performed immunofluorescence staining to analyse the expression of other components of the adherens junction, E-cadherin and β-catenin. At E13.5, β-catenin was expressed throughout the tooth germ epithelium, whereas E-cadherin exhibited stronger expression in a region anterior to the EK, reminiscent of E-cadherin expression in the molar, which is also absent in the EK [37] . After deletion of Ctnna1 , although the expression of β-catenin was unchanged, E-cadherin was upregulated in the presumptive EK region ( Supplementary Fig. 5i–l ). We next examined actin organization, as αE-catenin binds the actin filaments to the adherens junction. This was achieved by crossing the K14 GFP-actin allele [38] , which encodes a GFP–actin fusion protein, into the Ctnna1 cKO . Whereas actin was organized properly and constriction was visible at the apical side of the control basal cells ( Supplementary Fig. 5m,n ), this was lost in the Ctnna1 cKO ( Supplementary Fig. 5o,p ), potentially underlying the adhesion phenotype we observed. Importantly, the reduced adhesion seen in Ctnna1 cKO is unlikely to be the main cause of the EK phenotype we have observed, as similar disruption in cell–cell adhesion in K14 Cre ; Cdh1 fl/+ ; Ctnnd1 fl/fl , where one copy of Cdh1 (encoding E-cadherin) and both copies of Ctnnd1 (encoding p120-catenin) were deleted in the dental epithelium, did not affect EK formation, as evidenced by the robust p21 expression in these mutants ( Supplementary Fig. 6 ). Altogether, these data demonstrate that deletion of Ctnna1 in the tooth germ epithelium leads to severe defects in incisor morphogenesis, and its role in EK formation is independent of its involvement in cell–cell adhesion. αE-catenin is required for mesenchymal condensation It is thought that the EK functions as a signalling centre that provides both survival and instructive signals to the underlying mesenchyme, which in turn signals back to the epithelium for proper morphogenesis [7] . As the EK failed to form in the Ctnna1 cKO epithelium, we next set out to determine the effects of this failure on the dental mesenchyme. To that end, we performed in situ hybridization to examine the expression of Pax9 , Msx1 , Bmp4 and Fgf3 , which mark the dental mesenchyme. We found that at E13.5, as previously reported [24] , [26] , [39] , [40] , Bmp4 and Fgf3 are expressed in both the mesenchyme and the EK, while Pax9 and Msx1 are only present in the mesenchyme ( Figs 1j and 5a,c ). In the absence of αE-catenin, Pax9 and Msx1 expression was downregulated in the mesenchyme ( Fig. 5b,d ), and the size of the Bmp4 - and Fgf3 -expressing domains was reduced in the mesenchyme ( Fig. 1j ). 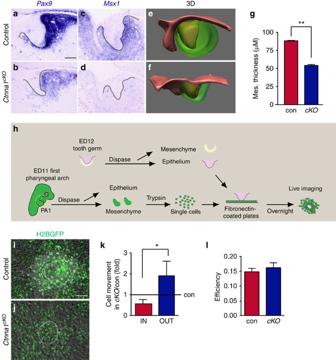Figure 5: αE-catenin is required for the epithelium-induced mesenchymal condensation during incisor development. (a–d)In situhybridization forPax9andMsx1in control andCtnna1cKO. In control embryos,Pax9andMsx1are expressed in the mesenchyme of the tooth germ at E13.5. InCtnna1cKO, the expression of these genes is reduced or absent. (e,f) 3D reconstruction of control andCtnna1cKOtooth germs at E13.5 (epithelium is red and mesenchyme is green). The thickness of the mesenchyme is reduced in the absence of αE-catenin. (g) Quantification of thickness of the condensed mesenchyme around the incisor dental epithelium at E13.5 (mean±s.e.m.,n=3,P<0.01). (h) Schematic illustration of thein vitrocondensation assay. ED, embryonic day; PA, pharyngeal arch. (i,j) H2B-GFP labelled wild-type mesenchymal cells robustly condense around the dissected control epitheliumin vitro(i) but fail to condense around theCtnna1cKOepithelium (j). White circles mark the position of GFP-negative epithelium. (k) Quantification of GFP-positive mesenchymal cells moving towards (IN) or away from (OUT) the epithelium showsCtnna1cKOepithelium is unable to retain mesenchymal cells in a condensed state (mean±s.e.m.,n=4 in control,n=3 inCtnna1cKO,P<0.05). (l) The efficiency of mesenchymal cell movement (displacement over distance travelled) is not affected by αE-catenin deletion (mean±s.e.m.,n=4 in control,n=3 inCtnna1cKO,P>0.05). All quantifications are analysed by using Student’st-test. *P<0.05, **P<0.01. Dotted lines outline the epithelium of the incisor tooth germ. Scale bar, 100 μm (a–d,i,j). Figure 5: αE-catenin is required for the epithelium-induced mesenchymal condensation during incisor development. ( a – d ) In situ hybridization for Pax9 and Msx1 in control and Ctnna1 cKO . In control embryos, Pax9 and Msx1 are expressed in the mesenchyme of the tooth germ at E13.5. In Ctnna1 cKO , the expression of these genes is reduced or absent. ( e , f ) 3D reconstruction of control and Ctnna1 cKO tooth germs at E13.5 (epithelium is red and mesenchyme is green). The thickness of the mesenchyme is reduced in the absence of αE-catenin. ( g ) Quantification of thickness of the condensed mesenchyme around the incisor dental epithelium at E13.5 (mean±s.e.m., n =3, P <0.01). ( h ) Schematic illustration of the in vitro condensation assay. ED, embryonic day; PA, pharyngeal arch. ( i , j ) H2B-GFP labelled wild-type mesenchymal cells robustly condense around the dissected control epithelium in vitro ( i ) but fail to condense around the Ctnna1 cKO epithelium ( j ). White circles mark the position of GFP-negative epithelium. ( k ) Quantification of GFP-positive mesenchymal cells moving towards (IN) or away from (OUT) the epithelium shows Ctnna1 cKO epithelium is unable to retain mesenchymal cells in a condensed state (mean±s.e.m., n =4 in control, n =3 in Ctnna1 cKO , P <0.05). ( l ) The efficiency of mesenchymal cell movement (displacement over distance travelled) is not affected by αE-catenin deletion (mean±s.e.m., n =4 in control, n =3 in Ctnna1 cKO , P >0.05). All quantifications are analysed by using Student’s t -test. * P <0.05, ** P <0.01. Dotted lines outline the epithelium of the incisor tooth germ. Scale bar, 100 μm ( a – d , i , j ). Full size image We next utilized Ctnna1 mutants to ask about roles of the EK in regulating the underlying mesenchyme. As the dental epithelium invaginates, dental mesenchymal cells begin to pack tightly around the growing epithelium [41] . Because the expression of Pax9 and Msx1 reflects this process [42] , [43] , [44] , their downregulation potentially indicates perturbed mesenchymal condensation [45] . We therefore compared the thickness of the condensed mesenchyme between control and Ctnna1 cKO tooth germs ( Supplementary Fig. 7 ) at E13.5, which showed that the mutant mesenchyme was 1.6 times thinner than the control mesenchyme ( Fig. 5e-g ). To confirm that this effect in the mesenchyme was due to defects in the epithelium, we performed an in vitro assay based on previous reports showing that isolated molar dental epithelium can induce mesenchymal cells from the first pharyngeal arch to condense [43] . Using this approach, control or Ctnna1 cKO epithelium was grafted onto dissociated control mesenchymal cells that were collected from embryos expressing Histone 2B-GFP (CAG-H2B-GFP), which allowed direct visualization and tracking of each mesenchymal cell using time lapse microscopy ( Fig. 5h ). Whereas control epithelium was able to induce robust mesenchymal condensation, GFP (green fluorescent protein)-positive cells remained scattered in the presence of Ctnna1 cKO incisor epithelium ( Fig. 5i,j ). By tracking individual cells, we found that more cells moved away from than migrated towards the mutant epithelium compared to the control ( Fig. 5k and Supplementary Movies 1–4 ). Thus, the Ctnna1 cKO epithelium did not attract mesenchymal cells as well as control epithelium, most likely as a result of the absence of the EK, which secrets a range of signalling molecules. Interestingly, the efficiency of cell movement, as defined by total displacement over total distance travelled, was unaffected ( Fig. 5l ), suggesting that the ability of mesenchymal cells to move is intrinsic and that signals from the EK provide directional cues to maintain continued mesenchymal condensation. Deletion of Yap / Taz in Ctnna1 mutants restores EK formation The above findings led us to hypothesize that a principal function of αE-catenin during incisor morphogenesis is to inhibit the transcriptional activity of YAP to suppress cell proliferation and promote EK formation and maintenance. As expression of constitutively active YAP did not fully repress p21 expression and EK formation, we suspected that additional factors, such as the YAP homologue TAZ, may be required to regulate EK formation. Similar to YAP, TAZ localization can be regulated by αE-catenin [46] . We therefore set out to test the hypothesis that combined deletion of Yap and Taz in the Ctnna1 cKO mutants would rescue the αE-catenin mutant phenotype. To that end, we generated K14 Cre ; Ctnna1 cKO ; Yap cKO ; Taz cKO triple mutants to analyse tooth germ morphology, cell proliferation and EK formation. Immunostaining of YAP showed effective removal of the protein in these mutants ( Supplementary Fig. 8a–d ). Interestingly, deletion of just Yap and Taz using K14 Cre did not have a marked effect on the morphology of the developing incisor, and the EK was fully formed ( Supplementary Fig. 9 ), indicating that compensatory mechanisms can support cellular proliferation in the absence of Yap and Taz . Remarkably, however, the K14 Cre ; Ctnna1 cKO ; Yap cKO ; Taz cKO triple mutants exhibited a tooth germ that had a comparable depth of invagination as the control at E13.5, although the width of the mutants remained decreased ( Fig. 6a–c ). Importantly, the Ki67-negative region in the triple mutants was re-established at the posterior side of the basal layer ( Fig. 6d–g and compare with Fig. 1d,e ), and p21-positive cells were again detected in this region ( Fig. 6h–l and compare Fig. 6j,k with Fig. 1g ). In situ hybridization showed that Shh was expressed in the presumptive EK region ( Fig. 6m,n ), which demonstrated that combined deletion of Yap and Taz rescued not only the cell biological features but also the molecular signals in the Ctnna1 cKO EK. 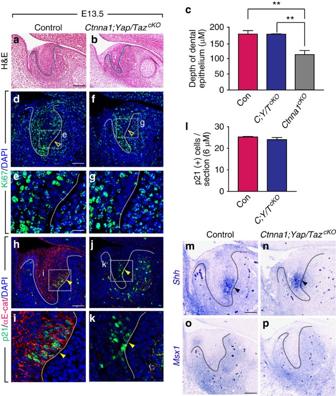Figure 6: αE-catenin regulates enamel knot formation and tooth germ invagination by controlling YAP/TAZ activity during tooth development. (a,b) H&E staining of E13.5 tooth germ shows that double deletion ofYap/Tazin theCtnna1cKOdental epithelium is able to rescue the invagination defect seen inCtnna1cKO. (c) Quantification of the depth of invaginated tooth germ in control, triple knockouts andCtnna1cKOat E13.5 (mean±s.e.m.,n=3,P<0.01). (d–g) Deletion ofYap/TazinCtnna1cKOrestores the non-proliferating zone at the posterior region of the tooth germ, as assessed by Ki67 staining, indicating the formation of the EK (open yellow arrowheads). (h–k) p21 staining confirms that deletion ofYap/TazinCtnna1cKOreestablishes a non-proliferating zone, indicating the formation of the EK in the tooth germ (yellow arrowheads). (l) Quantification of the number of p21-positive cells per section in control and triple knockout tooth germs (mean±s.e.m.,n=3,P>0.05). (m,n)Shhexpression at the posterior region of the tooth germ epithelium is rescued onYap/Tazdeletion in theCtnna1cKO(dark arrowheads). (o,p) Expression of the mesenchymal gene,Msx1,is rescued in the dental mesenchyme at E13.5 after deletion ofYap/TazinCtnna1cKOin the tooth germ. All quantifications are analysed by using Student’st-test. *P<0.05, **P<0.01. Dotted lines outline the epithelium of the incisor tooth germ. Scale bar, 100 μm (a,b); 50 μm (d,f,h,j,m–p); 8 μm (e,g,i,k). Figure 6: αE-catenin regulates enamel knot formation and tooth germ invagination by controlling YAP/TAZ activity during tooth development. ( a , b ) H&E staining of E13.5 tooth germ shows that double deletion of Yap / Taz in the Ctnna1 cKO dental epithelium is able to rescue the invagination defect seen in Ctnna1 cKO . ( c ) Quantification of the depth of invaginated tooth germ in control, triple knockouts and Ctnna1 cKO at E13.5 (mean±s.e.m., n =3, P <0.01). ( d – g ) Deletion of Yap / Taz in Ctnna1 cKO restores the non-proliferating zone at the posterior region of the tooth germ, as assessed by Ki67 staining, indicating the formation of the EK (open yellow arrowheads). ( h – k ) p21 staining confirms that deletion of Yap / Taz in Ctnna1 cKO reestablishes a non-proliferating zone, indicating the formation of the EK in the tooth germ (yellow arrowheads). ( l ) Quantification of the number of p21-positive cells per section in control and triple knockout tooth germs (mean±s.e.m., n =3, P >0.05). ( m , n ) Shh expression at the posterior region of the tooth germ epithelium is rescued on Yap/Taz deletion in the Ctnna1 cKO (dark arrowheads). ( o , p ) Expression of the mesenchymal gene, Msx1, is rescued in the dental mesenchyme at E13.5 after deletion of Yap / Taz in Ctnna1 cKO in the tooth germ. All quantifications are analysed by using Student’s t -test. * P <0.05, ** P <0.01. Dotted lines outline the epithelium of the incisor tooth germ. Scale bar, 100 μm ( a , b ); 50 μm ( d , f , h , j , m – p ); 8 μm ( e , g , i , k ). Full size image Next, we examined whether restoration of the EK in the triple mutants rescued the mesenchymal defect in Ctnna1 cKO . In situ hybridization showed that Msx1 expression was recovered in the mesenchyme to a level that was comparable to that in control ( Fig. 6o,p ), suggesting that the epithelial–mesenchymal feedback loop was re-established. Strikingly, histological analysis at E14.5 showed that the tooth germ in the triple mutants invaginated further and developed to cap stage ( Fig. 7a,b ). This was in stark contrast to the Ctnna1 cKO , where dental epithelium could barely be detected at this stage (compare Fig. 7b with Fig. 4h ). p21 staining also showed that the EK was maintained at E14.5 after deletion of Yap / Taz in the Ctnna1 cKO ( Fig. 7c–f ). Interestingly, disruptions were still apparent in sections of the triple mutants ( Fig. 7b ), providing further evidence that adhesive functions of αE-catenin during tooth development are separable from its role in EK formation, which involves the regulation of YAP/TAZ signalling. In this context, YAP appeared to play a more prominent role than TAZ, as Ctnna1 cKO ; Yap cKO ; Taz het tooth germs continued to invaginate at E16.5 ( Supplementary Fig. 8g,h ) and Ctnna1 cKO ; Yap het ; Taz cKO failed to do so ( Supplementary Fig. 8e,f ). 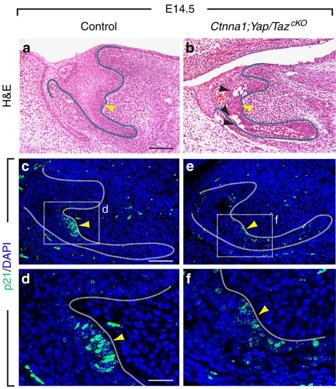Figure 7: The αE-catenin-YAP/TAZ signalling axis is required for further tooth germ invagination and development. (a,b) H&E staining of E14.5 tooth germ shows that theCtnna1cKOtooth germs passes the bud stage and progress to the cap stage after deletion ofYap/Taz. Black arrowheads mark tears within the tissue and yellow arrowheads mark EK. (c–f) p21-expressing cells (yellow arrowheads) are maintained at E14.5 in theCtnna1cKOtooth germ after deletion ofYap/Taz. Scale bar, 100 μm (a,b,c,e); 25 μm (d,f). Figure 7: The αE-catenin-YAP/TAZ signalling axis is required for further tooth germ invagination and development. ( a , b ) H&E staining of E14.5 tooth germ shows that the Ctnna1 cKO tooth germs passes the bud stage and progress to the cap stage after deletion of Yap / Taz . Black arrowheads mark tears within the tissue and yellow arrowheads mark EK. ( c – f ) p21-expressing cells (yellow arrowheads) are maintained at E14.5 in the Ctnna1 cKO tooth germ after deletion of Yap / Taz . Scale bar, 100 μm ( a , b , c , e ); 25 μm ( d , f ). Full size image A central event during tooth development is the formation of the EK, during which a group of proliferating cells exit the cell cycle, become densely packed at the posterior side of the epithelium, and begin to express an array of signalling molecules. However, the processes that regulate EK formation remain a mystery. Our observation that EK cells are devoid of nuclear YAP suggested that an active mechanism may be in place to regulate its localization and thus controls cell proliferation and EK formation. This was demonstrated through our conditional deletion of αE-catenin in the incisor epithelium. In the absence of αE-catenin, YAP accumulated in the nucleus of cells in the presumptive EK region, which continued to proliferate and failed to express the cell cycle inhibitor p21 and other EK markers, including Shh , Bmp4 and Fgf3 . Thus, the loss of Ctnna1 results in the complete absence of the EK. Importantly, this phenotype is due to the increased nuclear accumulation of YAP that acts cell-autonomously within the EK region, as mutants with EK-specific deletion of Lats1/2 failed to maintain the EK. This change in YAP activity accounts for the ectopic proliferation we observed, as expression of a constitutively active YAP ( Yap S127A ) or deletion of Lats1 / 2 -induced YAP nuclear localization and was sufficient to drive proliferation in the EK as well as downregulate p21 expression. It is therefore paradoxical at first glance that Ctnna1 mutant tooth germs are smaller than the control, despite increased proliferation in the EK. However, as the EK is a relatively small structure within the developing tooth, and cell proliferation is unchanged in the rest of the tissue, the increase in proliferation within the EK is not sufficient to compensate for loss of EK function in terms of the contribution to overall size. It should also be noted that the extent of inhibition of nuclear YAP by αE-catenin is different between EK and non-EK epithelial cells, suggesting that additional mechanisms must exist to either further restrict YAP in the cytoplasm in the EK or promote nuclear YAP accumulation in the non-EK cells. Interestingly, YAP and TAZ are dispensable for tooth germ invagination up to the bell stage ( Supplementary Fig. 9 ) [47] , indicating that additional mechanism(s) may be in place to compensate for their functions, and further studies are required to examine the role of YAP/TAZ in the non-EK epithelium. Our finding that nuclear YAP affects EK formation in the incisor is concordant with a recent paper that also utilized Yap S127A to study YAP function in the developing molar. In that paper, Shh expression in the presumptive EK region was similarly inhibited by the constitutively active YAP. Interestingly, an ectopic EK was reported in the molar in this paper; however, this finding is highly variable and occurs only on certain genetic backgrounds (X.-P. Wang, personal communication). We examined K14 Cre ;Yap S127A molars in our embryos and found that, in contrast to the earlier report, EK formation was inhibited without the induction of an ectopic EK ( Supplementary Fig. 2k–t ). Given the dependence on genetic background, the difference between our findings and the previous report are likely caused by the use of mice with different genetic backgrounds. To our knowledge, the Ctnna1 cKO is the first mutation shown to affect all aspects of EK formation, including cessation of cell proliferation and the production of signalling molecules. For example, in the downless ( Edar ) or tabby ( Eda ) mutant molars, although the EK forms and expresses p21 as well as Shh , Fgf4 and Bmp4 , the organization and the shape of the EK are dramatically altered [48] . In Lef1 −/− embryos, the EK is formed, as evidenced by the expression of p21, but key signalling molecules, such as Shh , Fgf3 and Fgf4 , are not expressed [49] . Therefore, αE-catenin may function upstream of these genes to first establish a group of non-proliferating cells, which are further regulated by EDA/EDAR and LEF1. Signals from the condensing dental mesenchyme such as BMP4 are also important for the establishment of the EK. By means of bead implantation, BMP4 was shown to be capable of inducing p21 expression [5] , and in Msx1 null mice, where Bmp4 expression is abrogated, cells in the presumptive EK region continue to proliferate, exhibiting a cell division phenotype similar to Ctnna1 cKO (ref. 50 ). Thus, αE-catenin may function within the epithelium in conjunction with BMP4 to regulate p21 expression and the cell cycle during formation of the EK. The disappearance of the EK in αE-catenin mutants presented an opportunity to test the functional requirement of the EK during odontogenesis. Since the discovery many years ago that the EK expresses an array of signalling molecules, it has been widely held that this structure acts as a signalling centre, guiding the development of the tooth. This notion is supported by several classical bead implantation experiments demonstrating that molecules secreted from the EK, such as FGFs, are sufficient to induce cell proliferation in both the non-EK epithelium and the mesenchyme, providing a mechanism for regulation of epithelial folding and the transition from the bud to the cap stage [8] , [51] . Similar experimental approaches have also been used to show that EK factors can induce expression of mesenchymal genes such as Runx2 (ref. 52 ). However, these gain-of-function studies did not explicitly test the functional requirement of the EK. Experiments using global gene inactivation, where the gene of interest is deleted in the entire animal, also could not determine whether the phenotypes were caused by the lack of the EK or by altered mesenchymal development. Here we show that absence of the EK as a result of epithelial deletion of Ctnna1 leads to failure of the dental mesenchyme to condense and express markers associated with condensation, such as Pax9 and Msx1 , as well as signalling molecules, such as Bmp4 and Fgf3 , which are important for odontogenesis and the regulation of the reciprocal epithelial–mesenchymal signalling pathways. This is similar to the Lef1 null mice, where LEF1 is required to induce Fgf3 expression in the mesenchyme through activation of epithelial FGF4 in molars. FGF3 in turn signals the epithelium to further regulate its development [49] . In Fgfr2(IIIb) −/− embryos, the molar tooth germs do not develop normally and fail to progress beyond the cap stage due to the decreased dental epithelial cell proliferation and loss of Fgf3 / 4 and Bmp4 expression in the EK [53] , [54] . Altogether, these results, along with our findings, show that the interaction between the EK and the mesenchyme by means of FGF and BMP signalling are important in maintaining mesenchymal condensation and proper epithelial cell proliferation and invagination. However, there remains the possibility that the mesenchymal phenotypes we have observed were a result of defects in the Ctnna1 non-EK epithelium, as currently there are no tools available to specifically disrupt the EK function before its formation. Our finding that YAP functions downstream of αE-catenin mirrors what has been observed in the skin, where expression of Yap S127A causes hyperproliferation, and deletion of Ctnna1 leads to increased nuclear YAP [17] . However, in contrast to observations made in the skin or during liver repair [12] , [17] , we did not observe hyperplasia and tumour formation in the tooth germ as a result of Ctnna1 deletion, but rather perturbed tissue morphogenesis due to failed cell cycle arrest and EK formation. These data thus suggest that the αE-catenin–YAP signalling axis is important both during embryonic development and adult tissue homeostasis, despite having distinct phenotypic outputs. However, how αE-catenin regulates YAP localization remains unclear. In the epidermis, 14-3-3 functions as an intermediate that connects αE-catenin to YAP and maintains YAP cytoplasmic localization in a LATS1/2- and MST1/2-independent manner [17] . αE-catenin further inhibits YAP activity by attenuating SRC function, which phosphorylates Y341/357/394 of YAP to promote YAP nuclear localization and transcriptional activity [55] . However, in other contexts, αE-catenin does seem to intersect with the Hippo core pathway. The LIM protein, Ajuba, can interact with αE-catenin and has been shown to interact with LATS1 and inhibit YAP phosphorylation [56] , [57] . Recently, it was also found in the epidermis that αE-catenin interacts with the neurofibromatosis type 2 (NF2) tumour suppressor, an upstream molecule in the Hippo pathway that bridges αE-catenin to PAR3 (ref. 58 ). Deletion of NF2 in the epidermis phenocopies αE-catenin null phenotypes. PAR3 itself can activate TAZ activity by inducing LATS1 dephosphorylation and inhibition through protein phosphatase 1 (PP1) interaction [59] . In the incisor tooth germ, we found that αE-catenin is required to maintain PAR3 apical localization and cell polarity, which in turn is critical for regulating YAP localization. This finding is consistent with previous reports in both Drosophila and mice that proper polarization of cells is required for correct YAP localization [30] , [31] . In addition, as deletion of Lats1/2 in the incisor epithelium induces nuclear YAP, the αE-catenin/PAR3 axis could potentially act upstream or in parallel of LATS1/2 to regulate YAP localization in the EK. Altogether, these results establish that αE-catenin is essential for normal tissue homeostasis via restriction of YAP in the cytoplasm through at least two distinct mechanisms. We next wanted to ask whether the increase in nuclear YAP is the main cause to the phenotypes observed. To tackle this question, we directly tested whether the increase in nuclear YAP and/or TAZ is required for the manifestation of the loss of αE-catenin by deleting both Yap and Taz in the Ctnna1 mutants. To our knowledge, this was the first attempted in vivo genetic rescue of a Ctnna1 cKO phenotype by deletion of Yap/Taz . Remarkably, the removal of both YAP and TAZ in the Ctnna1 mutants not only restored the EK structure and its function but also enabled the tooth germ to continue invaginating. This leads us to conclude that during tooth development, αE-catenin facilitates the formation of the EK by restricting YAP/TAZ in the cytoplasm, permitting the cells to exit the cell cycle and become specialized for signal production. One question that will be of great future interest is to further dissect the cell adhesion versus signalling functions of αE-catenin in formation of the EK. It is possible that during EK formation the adhesive function of αE-catenin is involved in the initial process of cell condensation, and that the protein subsequently has a second function of stopping proliferation based on regulation of YAP/TAZ. The rescue of tooth invagination in the K14 Cre ; Ctnna1 fl/fl ; Yap fl/fl ; Taz fl/fl triple mutants indicates that the cell adhesive function is not required for formation of the EK and progression to the cap stage, suggesting that other molecules could be involved in the regulation of cell condensation during EK formation. Interestingly, K14 Cre ; Cdh1 fl/+ ; Ctnnd1 fl/fl mutant embryos exhibited cell adhesion defects in the tooth germ, but had otherwise normal EK formation and tooth development ( Supplementary Fig. 6 ). These data support the notion that several aspects of early odontogenesis, including EK formation, epithelial invagination and mesenchymal condensation after lamina stage, are independent of cadherin mediated cell–cell adhesion, and instead rely on other mechanisms, such as correct maintenance of cell polarity and signal regulation of YAP. Signalling centres are the chief guiding force for the patterning and formation of many organs during development. However, the molecular and cellular mechanism underlying their formation remains less understood. Many signalling centres, such as the AER, floor plate and isthmus, have much reduced cell proliferation in comparison with the neighbouring cells [11] , [60] . This observation suggests that perhaps similar mechanisms are involved in formation of these signalling centres by causing cells to exit the cell cycle before becoming specialized in signal production. During formation of the EK, we have identified αE-catenin-dependent YAP/TAZ inhibition as a critical process for cells to commence the expression of p21 and cease proliferating. Interestingly, several signalling centres we have examined (AER, floor plate and isthmus) all express αE-catenin ( Supplementary Fig. 1t–x ) and have reduced nuclear YAP staining, low Ki67 labelling, and high p21 expression ( Supplementary Fig. 1a–r ). While this is a correlative observation, we suggest that some aspects of the mechanistic regulation of EK formation exist in the development of other signalling centres, which may also require αE-catenin to actively restrain nuclear YAP/TAZ accumulation and proliferation, allowing cell differentiation of a group of signal-producing cells. Mouse lines and induction of alleles K14-Cre (ref. 28 ), K14-actin-GFP (ref. 38 ), CAG-H2B-EGFP (ref. 61 ), Yap S127A (ref. 17 ), Shh CreER (ref. 62 ), Axin2 CreER (ref. 63 ) and conditional alleles of Ctnna1 (ref. 29 ), Lats1 and Lats2 (refs 64 , 65 ), Cdh1 (ref. 66 ), Ctnnd1 (ref. 67 ), Yap and Taz [68] , [69] were maintained and genotyped as previously reported. The mice maintained on mixed genetic backgrounds as a result of breeding between different lines. Age-matched littermates were used as controls in all cases, and both male and female embryos were included in all experiments. When Shh CreER or Axin2 CreER mice were used, tamoxifen was delivered to the pregnant females through intraperitoneal injection at stages indicated within the text. Activation of Yap S127A was achieved through provision of doxycycline in food starting at E9.5. All experiments involving mice were approved by the Institutional Animal Care and Use Committee of the University of California, San Francisco (protocol #AN099613). Tissue preparation and histological analysis E12.5 to E16.5 embryos were fixed with 4% paraformaldehyde (PFA) in PBS overnight at 4 °C. Embryos were embedded in paraffin. Sections were cut at 6 μm and stained with H&E using standard methods. Immunofluorescence staining For immunofluorescence, paraffin sections were rehydrated, and antigen retrieval was performed with citrate buffer containing 2 mM EDTA, 0.05% Tween 20 in a pressure cooker. Antibodies and dilutions used were as follows: αE-catenin (mouse, 1:500; BD Transduction Laboratories), β-catenin (rabbit, 1:1,000; Abcam), BrdU (rat, 1:500; Invitrogen), Ki67 (rat, 1:100; DAKO), GFP (rabbit, 1:1,000; Abcam), p21 (mouse, 1:500; BD Transduction Laboratories), YAP (rabbit, 1:100; Cell Signalling), and pYAP (rabbit, 1:100; Cell Signalling), E-cadherin (rat, 1:1,000; Zymed), Scribble (goat, 1:100; Cell signalling), PAR3 (rabbit, 1:500; Millipore). Secondary antibodies were coupled to Alexa 488, Alexa 555 (Invitrogen), or Biotin (Vector). TSA kit (PerkinElmer) was used for signal amplification for p21, YAP and pYAP detection. Nuclear counterstaining was performed with DAPI (Invitrogen), and all images were acquired using a Leica-TCS SP5 confocal microscope. In situ hybridization Sections (6 μm) were prepared and RNA in situ hybridization was performed on tissue sections using digoxigenin-labelled probes according to standard protocols. Alkaline phosphatase activity was detected on tissue sections using BM Purple staining solution (Roche) after overnight incubation in alkaline phosphatase buffer. Brightfield images were obtained using a Leica DFC 500 camera with a Leica DM 5000B microscope. 3D analysis of embryonic incisors The epithelium and mesenchyme were outlined from 30 to 60 consecutive 4-μm-thick sagittal sections ( n =3 animals per genotype). BioVis software ( http://www.biovis3d.com ) was used to generate 3D reconstructions. Incisor explant culture Lower mandibles were dissected out from E12.5 embryos and tongues were bladed away with fine needle in cold media. Mandibles were seeded into matrigel (20 μl) supplemented with 10 μM of Gö 6983 or DMSO control and laid into the cell insert with 350 μl of complete DMEM in the bottom. The complete DMEM was similarly supplemented with 10 μM of Gö 6983 (Selleckchem) or DMSO. Tissues were cultured for 72 h with changing of media every day. After 72 h, tissues were harvested and fixed with 4% PFA. Tissues were processed for paraffin section and the middle three sections were stained with YAP antibody to visualize its localization. Lentivirus infection of primary dental epithelial cells Dental epithelial cells from E12.5 tooth germs were infected using ∼ 25 μl of lentiviral supernatant (control shRNA and Par3 shRNA, Santa Cruz Biotechnology) with 5 μg ml −1 polybrene. Infections were typically performed in 6-well plates seeded with 15,000 cells. 12 h after infection, the supernatant was removed and cells were cultured with new media. Two days following infection, cells were fixed with 2.5% PFA and stained with YAP antibody. Determination of the condensed mesenchymal region The condensed mesenchyme can be easily distinguished from the surrounding non-condensed mesenchyme by visually inspecting H&E staining and a clear border can be drawn between the two regions, similar to earlier observations [43] , [44] , [45] . To statistically verify that we had indeed demarcated the two mesenchymal regions, we measured and compared the degree of coherence (similarity in cell orientation of adjacent cells [70] ) within the condensed and non-condensed mesenchyme. Briefly, cell orientation angles were determined using ImageJ, and for each cell, the difference in cell orientation was calculated for cells within 50-pixels distance and used to derive the s.d. for this subset. This was repeated for all cells and an average of the s.d. was acquired for cells within the condensed and non-condensed mesenchyme. A Student’s t- test was then used to determine whether the coherence between these two regions was statistically distinct. In vitro condensation and live imaging For this assay, the published method [43] was used with slight modification. The first pharyngeal arch was dissected from CAG-H2B-EGFP E11 embryos and treated with Dispase II (2.4 U ml −1 ; Roche) at 37 °C for 13 min. After a 13-min incubation, 3 ml DMEM was added to stop digestion. The epithelium was removed and the dental mesenchyme was dissected out and incubated with 0.05% trypsin for 1 min, gently triturated several times, and 8 × 10 4 cells plated into 12-well fibronectin (Becton Dickinson)-coated glass bottom dishes (MatTek Corporation) in 400 μl DMEM supplemented with 10% fetal bovine serum. The media was changed the next day, and after 2 days of culturing, when the cells reached around 90% confluence, freshly isolated E12 dental epithelium from controls and Ctnna1 mutants were overlaid on top of the monolayer of GFP-positive mesenchymal cells and cultured for 48 h. For live imaging, after overnight incubation to let the epithelium adhere to the mesenchymal cells, images were acquired every 4 min for 24 h using a Leica LP5 confocal microscope. μCT imaging analysis Mandibles from E16.5 embryos were harvested and dehydrated through ethanol series to 70% ethanol. Samples were then soaked in phosphotungstic acid overnight to differentially stain soft tissues for μCT visualization using MicroXCT-200 (Xradia) with a spatial resolution of 0.5 μm. Images acquired were analysed using Avizo (VSG). Statistical analysis Data were reported as means±s.e.m. Unpaired Student’s t -test was performed where significance was indicated by two-tailed P values; * P <0.05, ** P <0.01 and *** P <0.001. Data availability The authors declare that the data supporting the findings of this study are available within the article and its Supplementary Information files. How to cite this article: Li, C.-Y. et al. αE-catenin inhibits YAP/TAZ activity to regulate signalling centre formation during tooth development. Nat. Commun. 7:12133 doi: 10.1038/ncomms12133 (2016).